Loss-of-function of inositol polyphosphate-4-phosphatase reversibly increases the severity of allergic airway inflammation Inositol polyphosphate phosphatases regulate the magnitude of phosphoinositide-3 kinase signalling output. Although inositol polyphosphate-4-phosphatase is known to regulate phosphoinositide-3 kinase signalling, little is known regarding its role in asthma pathogenesis. Here we show that modulation of inositol polyphosphate-4-phosphatase alters the severity of asthma. Allergic airway inflammation in mice led to calpain-mediated degradation of inositol polyphosphate-4-phosphatase. In allergic airway inflammation models, preventing inositol polyphosphate-4-phosphatase degradation by inhibiting calpain activity, or overexpression of inositol polyphosphate-4-phosphatase in mouse lungs, led to attenuation of the asthma phenotype. Conversely, knockdown of inositol polyphosphate-4-phosphatase severely aggravated the allergic airway inflammation and the asthma phenotype. Interestingly, inositol polyphosphate-4-phosphatase knockdown in lungs of naive mice led to spontaneous airway hyper-responsiveness, suggesting that inositol polyphosphate-4-phosphatase could be vital in maintaining the lung homeostasis. We suggest that inositol polyphosphate-4-phosphatase has an important role in modulating inflammatory response in asthma, and thus, uncover a new understanding of the complex interplay between inositol signalling and asthma, which could provide alternative strategies in asthma management. Phosphoinositide signalling, from phosphoinositide-3-kinase (PI3K) activation to Akt phosphorylation, critically regulates cellular functions, such as cell growth, differentiation, proliferation, survival and motility [1] . In response to growth factor stimuli, activation of PI(3)Ks leads to generation of PtdIns(3,4,5)P3 and PtdIns(3,4)P2 at the plasma membrane. The intracellular concentration of PtdIns(3,4,5)P3 is controlled by a 3-phosphatase known as phosphatase and tensin homologue (PTEN) [2] or by 5-phosphatases (SHIP) [3] , resulting in the production of PtdIns(4,5)P2 and PtdIns(3,4)P2, respectively. PtdIns(3,4)P2, in turn, gets degraded by inositol polyphosphate-4-phosphatase (INPP4) to form PtdIns(3)P [4] . Genotypic variations in type I INPP4 (INPP4A), which is a regulatory checkpoint in phosphoinositide signalling, have previously been shown to be associated with increased risk of asthma [5] , [6] .Although other phosphoinositide phosphatases, PTEN and SHIP, have been shown to importantly regulate T-cell activation [7] , [8] , suppress B-cell lymphoma [9] and have protective roles in allergic airway inflammation (AAI) [10] , [11] , the functional role of INPP4A, in this context, is not known. As PtdIns(3,4)P2, but not PtdIns(3,4,5)P3, potently activates Akt [12] , INPP4A effectively terminates the PI3K-Akt signalling cascade. Asthma is characterized by episodic bronchoconstriction due to airway inflammation, remodelling and hyper-responsiveness [13] . Metabolic origins of asthma in obese subjects with minimal inflammatory cell infiltrate are an active topic of research [14] . Current understanding and treatment of asthma focuses on inhibiting airway inflammation and constriction. Although this is largely effective, there are a substantial number of poor responders, particularly amongst those with either very high or very low inflammatory cells in sputum [15] . Exploration of novel downstream pathways [16] that may be common to inflammatory as well as non-inflammatory origins of asthma, is therefore of interest. Notably, activation of the PI3K-Akt pathway can induce airway smooth muscle proliferation [17] , platelet activation [18] , mast cell degranulation [19] , cytokine production in mast cells [20] and corticosteroid insensitivity in chronic respiratory diseases [21] . Lipid phosphatases such as INPP4A are regulatory checkpoints that control detrimental actions of the PI3K signalling in 3-phosphoinositide lipid network [22] . Loss of such regulatory checkpoints may be important for the development of the asthma phenotype, and their restoration may be of therapeutic interest. Considering that there is very little information on the role of INPP4A in asthma, in this report we demonstrate for the first time that AAI in mice leads to calpain-protease-mediated degradation of INPP4A in bronchial epithelium. Restoration of INPP4A by administration of the calpain inhibitor, calpeptin, alleviates asthma. Conversely, lung-specific knockdown of INPP4A by small interfering RNA (siRNA) induces spontaneous inflammation in mice, even in the absence of allergic sensitization, possibly by activating the PI3K-Akt pathway. In mice with experimental asthma, further knockdown of INPP4A by siRNA leads to a severe asthma phenotype, whereas overexpression of INPP4A reverses airway hyper-responsiveness (AHR) and airway inflammation in allergic mice. These links between a critical signalling pathway and asthma provides new understanding of the complex interplay between INPP4A and asthma, and provide hope for alternative strategies in asthma management. Loss of INPP4A in AAI An established mouse model of AAI was used ( Fig. 1a ). To investigate the function of INPP4A in AAI, we first examined the expression of INPP4A in lungs from normal and allergic mice. The allergic-inflamed lungs from mice with experimental asthma showed a significant reduction of INPP4A transcripts, protein levels and enzymatic activity ( Fig. 1b-d ). In normal mouse lungs, INPP4A was predominantly expressed in apical regions of bronchial epithelial cells, with markedly diminished expression during allergic inflammation ( Fig. 1e ). Fluorescence-activated cell sorting analysis of single-cell suspensions prepared from control and allergically inflamed lungs confirmed our observations ( Fig. 1f ). Further, INPP4A-expressing cytokeratin-positive cells (marker of epithelial cells) in single-cell suspensions from the lung were also decreased in allergic mice compared with control mice ( Fig. 1g ). 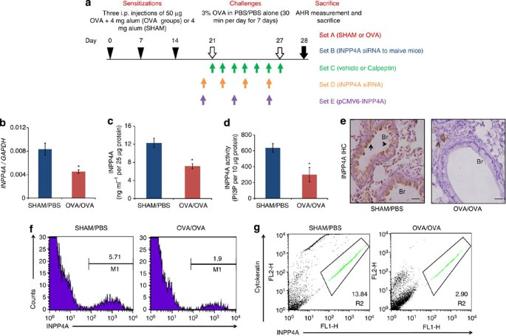Figure 1: Loss of INPP4A in acute allergic inflammation. (a) Experimental protocols for different AAI models as described in the Methods. (b) INPP4A mRNA levels, (c) protein levels and (d) enzymatic activity in lungs with (OVA/OVA) or without AAI (SHAM/PBS) are shown. (e) Immunohistochemical (IHC) staining for INPP4A in lung sections from mice with and without AAI. Brown colour indicates the positive expression. Representative photomicrographs from three independent experiments have been shown. Br, bronchus. Black arrows indicate the INPP4A positivity in bronchial epithelial cells. Scale bars equal 50 μM. (f) Representative flow cytometry histogram of INPP4A-stained cell population in the lung single-cell suspension of control and allergic mice. (g) INPP4A and cytokeratin double-positive cell population in control and allergic mice. Independent replicates were performed for all experiments (n=6 per group) and the data is shown as mean±s.e.m. throughout; *denoteP<0.05 versus SHAM/PBS. Significant differences between two selected groups were estimated using the unpaired Student'st-test. Figure 1: Loss of INPP4A in acute allergic inflammation. ( a ) Experimental protocols for different AAI models as described in the Methods. ( b ) INPP4A mRNA levels, ( c ) protein levels and ( d ) enzymatic activity in lungs with (OVA/OVA) or without AAI (SHAM/PBS) are shown. ( e ) Immunohistochemical (IHC) staining for INPP4A in lung sections from mice with and without AAI. Brown colour indicates the positive expression. Representative photomicrographs from three independent experiments have been shown. Br, bronchus. Black arrows indicate the INPP4A positivity in bronchial epithelial cells. Scale bars equal 50 μM. ( f ) Representative flow cytometry histogram of INPP4A-stained cell population in the lung single-cell suspension of control and allergic mice. ( g ) INPP4A and cytokeratin double-positive cell population in control and allergic mice. Independent replicates were performed for all experiments ( n =6 per group) and the data is shown as mean±s.e.m. throughout; *denote P <0.05 versus SHAM/PBS. Significant differences between two selected groups were estimated using the unpaired Student's t -test. Full size image Loss of INPP4A in interleukin-13 induced airway epithelial cells As we found a prominent expression of INPP4A in mouse lungs, we used human bronchial epithelial cells as a model system to examine the expression of INPP4A. As interleukin (IL)-13 is one of the pivotal cytokines involved in asthma pathogenesis, we induced BEAS-2B cells with IL-13 for various time periods and monitored the expression of INPP4A. INPP4A expression was reduced in human bronchial epithelial cells with IL-13 stimulation as time increased ( Fig. 2a,b ). A similar reduction in the expression of INPP4A was observed in primary-cultured airway epithelial cells induced with IL-13 ( Fig. 2c ). As calpains are previously known to degrade INPP4A in human platelets, to investigate the mechanism of degradation of INPP4A, we estimated calpain activity in IL-13-induced BEAS-2B extracts. We observed a sharp increase in calpain activity with IL-13 stimulation ( Fig. 2d ), which corresponds to the fall in the expression of INPP4A ( Fig. 2a ). 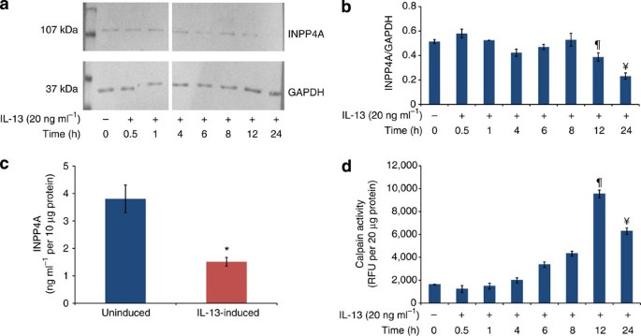Figure 2: Loss of INPP4A in IL-13-induced airway epithelial cells. (a) Western blot analysis of INPP4A and GAPDH in IL-13-induced BEAS-2B cells for various time periods and (b) their densitometric analysis. (c) Epithelial cells were isolated and cultured from murine airway and induced with IL-13 for 24 h. INPP4A protein levels were measured and results are expressed as ng ml−1per 10 μg protein. (d) Calpain activity in BEAS-2B cell lysates; RFU-relative fluorescence units. Data were mean±s.e.m. of three independent experiments. ¶ and ¥ denoteP<0.05 at 12 and 24 h, respectively, after IL-13 induction versus unstimulated BEAS-2B cells; and *denotesP<0.05 versus uninduced murine tracheal epithelial cells. Significant differences between two selected groups were estimated using the unpaired Student'st-test. Figure 2: Loss of INPP4A in IL-13-induced airway epithelial cells. ( a ) Western blot analysis of INPP4A and GAPDH in IL-13-induced BEAS-2B cells for various time periods and ( b ) their densitometric analysis. ( c ) Epithelial cells were isolated and cultured from murine airway and induced with IL-13 for 24 h. INPP4A protein levels were measured and results are expressed as ng ml −1 per 10 μg protein. ( d ) Calpain activity in BEAS-2B cell lysates; RFU-relative fluorescence units. Data were mean±s.e.m. of three independent experiments. ¶ and ¥ denote P <0.05 at 12 and 24 h, respectively, after IL-13 induction versus unstimulated BEAS-2B cells; and *denotes P <0.05 versus uninduced murine tracheal epithelial cells. Significant differences between two selected groups were estimated using the unpaired Student's t -test. Full size image Calpain-mediated degradation of INPP4A is vital for asthma A characteristic PEST sequence (a sequence rich in proline (P), glutamic acid (E), serine (S) and threonine (T) serves as proteolytic recognition sites for calpain) was observed in the murine INPP4A protein domain ( Fig. 3a ). Calpain activity was also found to be increased in allergically inflamed lungs compared with normal lungs, and pooled analysis of all samples ( n =24) showed that calpain activity and INPP4A activity were significantly negatively correlated ( Fig. 3b ), suggesting that calpain is primarily responsible for INPP4A degradation in AAI. Administration of a specific calpain inhibitor (calpeptin) to mice with AAI ( Fig. 1a ) reduced calpain activity ( Fig. 3c ), and restored INPP4A activity ( Fig. 3d ) and expression in allergically inflamed lungs ( Fig. 3e ). This was associated with marked improvement of the asthma phenotype, including AHR ( Fig. 3f ); inflammation score ( Fig. 3g ); airway inflammation ( Fig. 3h ), including bronchoalveolar lavage (BAL) fluid eosinophilia ( Supplementary Fig. S1a ); goblet cell metaplasia ( Fig. 3i ); sub-epithelial fibrosis ( Fig. 3j ); and inflammatory cytokine profile, including IL-4, IL-5, IL-13, transforming growth factor (TGF)-β1 and ova-specific immunonuglobulin E (IgE; Table 1 ). 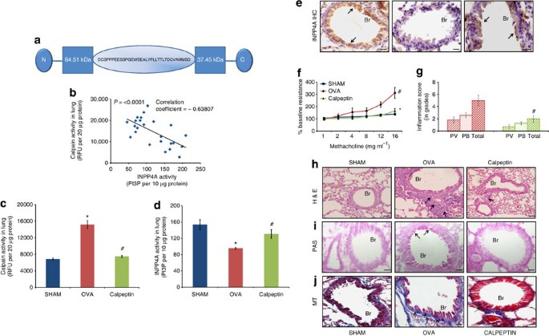Figure 3: Calpain-mediated degradation of INPP4A is important for allergic asthma. (a) Schematic diagram to show the calpain site of action (PEST sequence) in the INPP4A protein domain of mouse. (b) Correlation analysis of INPP4A activity (xaxis) with calpain activity (yaxis) is shown for mice with and without AAI. Effect of calpeptin on (c) calpain activity, (d) INPP4A activity, (e) INPP4A expression, (f) AHR, (g) inflammation score, (h) airway inflammation (haematoxylin and eosin (H&E) staining), (i) goblet cell metaplasia (periodic acid-Schiff (PAS) staining), and (j) sub-epithelial fibrosis (Masson's trichome (MT) staining) in murine model of AAI. Scale bars equal 50 μM. Br, bronchus. PV and PB denote perivascular and peribronchial inflammation, respectively. Black arrows, dashed arrows, lined arrows and dotted arrows denote INPP4A positivity, inflammatory cell infiltrate, mucus and collagen, respectively. SHAM, OVA and Calpeptin denote SHAM/PBS/VEH, OVA/OVA/VEH and OVA/OVA/Calpeptin, respectively. Data were mean±s.e.m. of three independent experiments (n=6 per group). *P<0.05 versus SHAM, #P<0.05 versus OVA. Significant differences between two selected groups were estimated using the unpaired Student'st-test. Figure 3: Calpain-mediated degradation of INPP4A is important for allergic asthma. ( a ) Schematic diagram to show the calpain site of action (PEST sequence) in the INPP4A protein domain of mouse. ( b ) Correlation analysis of INPP4A activity ( x axis) with calpain activity ( y axis) is shown for mice with and without AAI. Effect of calpeptin on ( c ) calpain activity, ( d ) INPP4A activity, ( e ) INPP4A expression, ( f ) AHR, ( g ) inflammation score, ( h ) airway inflammation (haematoxylin and eosin (H&E) staining), ( i ) goblet cell metaplasia (periodic acid-Schiff (PAS) staining), and ( j ) sub-epithelial fibrosis (Masson's trichome (MT) staining) in murine model of AAI. Scale bars equal 50 μM. Br, bronchus. PV and PB denote perivascular and peribronchial inflammation, respectively. Black arrows, dashed arrows, lined arrows and dotted arrows denote INPP4A positivity, inflammatory cell infiltrate, mucus and collagen, respectively. SHAM, OVA and Calpeptin denote SHAM/PBS/VEH, OVA/OVA/VEH and OVA/OVA/Calpeptin, respectively. Data were mean±s.e.m. of three independent experiments ( n =6 per group). * P <0.05 versus SHAM, # P <0.05 versus OVA. Significant differences between two selected groups were estimated using the unpaired Student's t -test. Full size image Table 1 Cytokine profile in different groups of mice. Full size table Loss of INPP4A induces asthma-like condition in naive mice Next, to determine whether the loss of INPP4A is sufficient to induce asthma-like condition, we treated naive mice without any allergen sensitization and challenge with inhaled INPP4A siRNA ( Fig. 4a ). The efficacy of INPP4A siRNA in downregulating INPP4A transcripts was confirmed by real-time PCR ( Fig. 4b ). Interestingly, naive mice treated with INPP4A siRNA developed characteristic AHR ( Fig. 4c ), similar to mice with allergic inflammation, but without the intense inflammatory cell infiltrate ( Fig. 4d , Supplementary Fig. S1b ). INPP4A siRNA-treated mice also showed a modest increase in mucin content ( Fig. 4e ) and collagen deposition ( Fig. 4f ). Notably, some mice showed low-grade spontaneous peribronchial inflammatory infiltrate, despite absence of any sensitization, challenge or infection. However, naive mice treated with scrambled siRNA did not show AHR or any other feature, confirming that this was specific to INPP4A knockdown. Moreover,increased activation of the PI3K-Akt signalling was observed in INPP4A siRNA-treated naive mice as measured by the levels of PDK1 ( Fig. 4g ), Akt kinase activity ( Fig. 4h ) and phospho-Akt ( Fig. 4i ), suggesting a critical role of INPP4A in maintaining the normal lung function. To investigate whether administration of siRNA in mice led to the non-specific induction of interferon (IFN)-α, IFN-β, IFN-γ and IL-12, we measured the levels of these cytokines in the lungs of siRNA-administered mice. Importantly, administration of siRNA to naive mice did not induce type-I IFN responses, such as release of IFN-α or IFN-β, or toll-like receptor-3-dependent upregulation of IFN-γ and IL-12 [23] ( Supplementary Fig. S2a–d ), excluding non-specific effects. 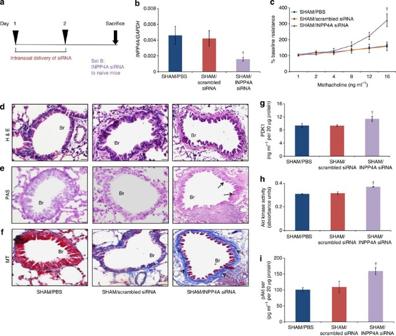Figure 4: Loss of INPP4A is sufficient to induce asthma-like condition in naive mice without any sensitization and challenge. (a) Experimental protocol (set B) for administration of siRNA in naive mice as described in Methods. (b) The relative expression of INPP4A transcripts in siRNA-administered murine lungs compared with normal lungs. †P<0.05 versus SHAM/Scrambled siRNA. Effect of scrambled or INPP4A siRNA on (c) AHR to methacholine challenge, (d) airway inflammation (haematoxylin and eosin (H&E) staining), (e) goblet cell metaplasia (periodic acid-Schiff (PAS) staining) and (f) sub-epithelial fibrosis (Masson's trichome (MT) staining) in lung sections, and (g) PDK1 levels, (h) Akt kinase activity and (i) cytosolic pAkt Ser in lungs of naive mice without AAI. Data were mean±s.e.m. of three independent experiments (n=6 per group). † denoteP<0.05 versus SHAM/Scrambled siRNA. Scale bars equal 50 μM. Br, bronchus. Lined arrows and dotted arrows denote mucus and collagen deposition, respectively.P-value was calculated using one tailedt-test. Figure 4: Loss of INPP4A is sufficient to induce asthma-like condition in naive mice without any sensitization and challenge. ( a ) Experimental protocol (set B) for administration of siRNA in naive mice as described in Methods. ( b ) The relative expression of INPP4A transcripts in siRNA-administered murine lungs compared with normal lungs. † P <0.05 versus SHAM/Scrambled siRNA. Effect of scrambled or INPP4A siRNA on ( c ) AHR to methacholine challenge, ( d ) airway inflammation (haematoxylin and eosin (H&E) staining), ( e ) goblet cell metaplasia (periodic acid-Schiff (PAS) staining) and ( f ) sub-epithelial fibrosis (Masson's trichome (MT) staining) in lung sections, and ( g ) PDK1 levels, ( h ) Akt kinase activity and ( i ) cytosolic pAkt Ser in lungs of naive mice without AAI. Data were mean±s.e.m. of three independent experiments ( n =6 per group). † denote P <0.05 versus SHAM/Scrambled siRNA. Scale bars equal 50 μM. Br, bronchus. Lined arrows and dotted arrows denote mucus and collagen deposition, respectively. P -value was calculated using one tailed t -test. Full size image INPP4A knockdown increases the severity of asthma To further confirm the pro-inflammatory and pro-asthma role of loss of INPP4A, we knocked down INPP4A in the murine model of AAI. Targeted knockdown of INPP4A in lungs by inhaled siRNA led to an increase in AHR ( Fig. 5a ), inflammation score ( Fig. 5b ) and airway inflammation ( Fig. 5c , Supplementary Fig. S3 ), Th2 cytokine profile, including IL-4, IL-5, IL-13, TGF-β1 and ova-specific IgE ( Table 1 ), and was associated with increased airway remodelling, including goblet cell metaplasia ( Fig. 5d ) and sub-epithelial fibrosis ( Fig. 5e ). Expression of INPP4A was not observed in INPP4A knockdown mice by immunohistochemistry ( Fig. 5f ). Knockdown of INPP4A led to increased activation of the PI3K-Akt pathway as evident by the increased levels of pAkt Ser, pAkt Thr, PDK1 and Akt kinase activity in INPP4A siRNA-treated mice with AAI ( Fig. 5g-j ). Similar to naive mice, siRNA delivery to mice with AAI did not induce typeI IFN response, such as release of IFN-α or IFN-β, or toll-like receptor-3-dependent upregulation of IFN-γ and IL-12 [23] ( Supplementary Fig. S4 a–d ). 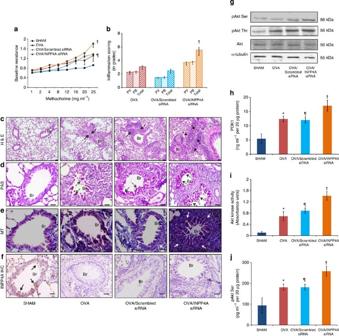Figure 5: Loss of INPP4A worsens asthmatic phenotype with increased activation of the PI3K-Akt pathway. Effect of INPP4A knockdown on (a) AHR to methacholine challenge, (b) inflammation score, (c) airway inflammation (haematoxylin and eosin (H&E) staining), (d) goblet cell metaplasia (periodic acid-Schiff (PAS) staining), (e) sub-epithelial fibrosis (Masson's trichome (MT) staining), (f) INPP4A expression, (g) expressions of pAkt Ser, pAkt Thr, Akt and α-tubulin, (h) levels of PDK1, (i) Akt kinase activity and (j) pAkt Ser in lungs of mice with AAI. Scale bars equal 50 μM. Br, bronchus. SHAM, OVA, OVA/Scrambled siRNA, OVA/INPP4A siRNA denote SHAM/PBS/VEH, OVA/OVA/VEH, OVA/OVA/Scrambled siRNA and OVA/OVA/INPP4A siRNA, respectively. Data were mean±s.e.m. of three independent experiments, (n=5 per group). *P<0.05 versus SHAM, ¶P<0.05 versus SHAM, and †P<0.05 versus Scrambled.P-value was calculated using unpaired Student'st-test. Black arrows, dashed arrows, lined arrows and white arrows denote INPP4A positivity, inflammatory cell infiltrate, mucus and collagen, respectively. Figure 5: Loss of INPP4A worsens asthmatic phenotype with increased activation of the PI3K-Akt pathway. Effect of INPP4A knockdown on ( a ) AHR to methacholine challenge, ( b ) inflammation score, ( c ) airway inflammation (haematoxylin and eosin (H&E) staining), ( d ) goblet cell metaplasia (periodic acid-Schiff (PAS) staining), ( e ) sub-epithelial fibrosis (Masson's trichome (MT) staining), ( f ) INPP4A expression, ( g ) expressions of pAkt Ser, pAkt Thr, Akt and α-tubulin, ( h ) levels of PDK1, ( i ) Akt kinase activity and ( j ) pAkt Ser in lungs of mice with AAI. Scale bars equal 50 μM. Br, bronchus. SHAM, OVA, OVA/Scrambled siRNA, OVA/INPP4A siRNA denote SHAM/PBS/VEH, OVA/OVA/VEH, OVA/OVA/Scrambled siRNA and OVA/OVA/INPP4A siRNA, respectively. Data were mean±s.e.m. of three independent experiments, ( n =5 per group). * P <0.05 versus SHAM, ¶ P <0.05 versus SHAM, and † P <0.05 versus Scrambled. P -value was calculated using unpaired Student's t -test. Black arrows, dashed arrows, lined arrows and white arrows denote INPP4A positivity, inflammatory cell infiltrate, mucus and collagen, respectively. Full size image Overexpression of INPP4A protects mice from asthma To better understand the protective role of INPP4A in asthma pathogenesis, we overexpressed INPP4A via intravenous administration of pCMV6-INPP4A, using in vivo -jetPEI in the murine model of AAI. Intravenous administration of plasmids complexed with in vivo -jetPEI has already been shown to effectively reach lungs ( Supplementary Fig. S5a–c ) [24] . Mice that received 50 μg pCMV6-INPP4A plasmid showed significant expression of INPP4A ( Fig. 6a , Supplementary Fig. S6 ) as compared with those mice that received 25 ìg plasmid, and hence, it was chosen for further experiments. As shown in Fig. 6b , INPP4A overexpression in allergic mice was associated with reduced AHR. Corresponding trends were observed in inflammation score ( Fig. 6c ). Histopathological analysis revealed that mice administered with 50 ìg pCMV6-INPP4A showed more INPP4A expression ( Fig. 6d ), a reduction in airway inflammation ( Fig. 6e , Supplementary Fig. S7 ), less effect on goblet cell metaplasia ( Fig. 6f ) and a significant reduction in collagen deposition ( Fig. 6g ). Interestingly, there was not much reduction in goblet cell metaplasia with INPP4A overexpression, possibly related to patchy overexpression ( Fig. 6f ).The increased IL-4, IL-5, TGF-β and IgE levels in the lung and sera of mice with AAI were significantly reduced by INPP4A overexpression ( Table 1 ). However, there was a marginal reduction in the levels of IL-13 with INPP4A overexpression ( P -value=0.0926 using unpaired Student's t -test). To determine whether the attenuation of the asthma phenotype with INPP4A overexpression correlates with decreased PI3K-Akt signalling, levels of PDK1 ( Fig. 6h ), Akt kinase activity ( Fig. 6i ) and phosphorylation of Akt ( Fig. 6j ) were measured. We observed potent alleviation of airway inflammation and asthma features with a significant suppression of the PI3K-Akt signalling in INPP4A-overexpressed lungs of mice with AAI ( Fig. 6h–j ). 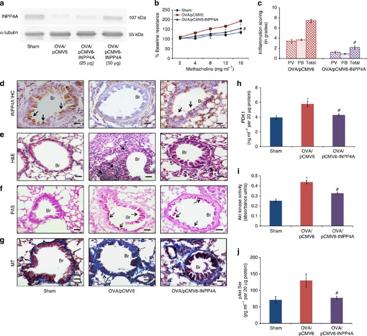Figure 6: Overexpression of INPP4A protects mice from asthma. (a) Western blot analysis of INPP4A in lungs of mice administered with INPP4A overexpression plasmid. Effect of INPP4A overexpression on (b) AHR to methacholine challenge, (c) inflammation score, (d) INPP4A immunolocalization in the lung, (e) airway inflammation (haematoxylin and eosin (H&E) staining), (f) goblet cell metaplasia (periodic acid-Schiff (PAS) staining), (g) sub-epithelial fibrosis (Masson's trichome (MT) staining), (h) Levels of PDK1, (i) Akt kinase activity and (j) cytosolic pAkt Ser in mice with AAI. Scale bars equal 50 μM. Br, bronchus. SHAM, OVA/pCMV6 and OVA/pCMV6-INPP4A denote SHAM/PBS/VEH, OVA/OVA/pCMV6 and OVA/OVA/pCMV6-INPP4A, respectively. Data were mean±s.e.m. of three independent experiments (n=5 per group). *P<0.05 versus SHAM, #P<0.05 versus OVA/pCMV6.P-value was calculated using one tailedt-test. Black arrows, dashed arrows, lined arrows and dotted arrows denote INPP4A positivity, inflammatory cell infiltrate, mucus and collagen, respectively. Figure 6: Overexpression of INPP4A protects mice from asthma. ( a ) Western blot analysis of INPP4A in lungs of mice administered with INPP4A overexpression plasmid. Effect of INPP4A overexpression on ( b ) AHR to methacholine challenge, ( c ) inflammation score, ( d ) INPP4A immunolocalization in the lung, ( e ) airway inflammation (haematoxylin and eosin (H&E) staining), ( f ) goblet cell metaplasia (periodic acid-Schiff (PAS) staining), ( g ) sub-epithelial fibrosis (Masson's trichome (MT) staining), ( h ) Levels of PDK1, ( i ) Akt kinase activity and ( j ) cytosolic pAkt Ser in mice with AAI. Scale bars equal 50 μM. Br, bronchus. SHAM, OVA/pCMV6 and OVA/pCMV6-INPP4A denote SHAM/PBS/VEH, OVA/OVA/pCMV6 and OVA/OVA/pCMV6-INPP4A, respectively. Data were mean±s.e.m. of three independent experiments ( n =5 per group). * P <0.05 versus SHAM, # P <0.05 versus OVA/pCMV6. P -value was calculated using one tailed t -test. Black arrows, dashed arrows, lined arrows and dotted arrows denote INPP4A positivity, inflammatory cell infiltrate, mucus and collagen, respectively. Full size image Although the roles of PTEN and SHIP, key negative regulators of the PI3K signalling pathway, in various inflammatory diseases, including airway inflammation and asthma, have been studied [25] , [26] , [27] , the role of another key phosphatase, INPP4A, has not yet been elucidated. Here we report for the first time that INPP4A is vital as a negative regulator of asthma pathogenesis, and reduced expression of INPP4A could lead to a severe asthma phenotype. Our study is unique in deciphering and reporting a correlation between expression of INPP4A and AAI. Our immunohistochemical analysis on tissue sections from normal and allergically inflamed mouse lungs revealed that INPP4A is predominantly expressed in bronchial epithelial cells, and that, its expression is reduced in allergically inflamed lungs. We confirmed our findings in vitro , where we observed that INPP4A is reduced by IL-13 induction of mouse primary respiratory epithelial cells and a human bronchial epithelial cell line. It has been previously reported that IL-13 induction in a human colonic epithelial cell line led to the accumulation of lipid products of PI3K, such as PtdIns(3,4)P2 and PtdIns(3,4,5)P3, which corroborates with the observation that INPP4A falls with IL-13 induction in human bronchial epithelial cells [28] . The mechanism of INPP4A degradation during allergic inflammation pertains to the increase in the activity of calpain. It has been shown that calpain degrades and inactivates INPP4A in human platelets on recognition of the PEST motif [29] . As PEST sequences are calpain protease target sites, and a characteristic PEST motif was also seen in mouse INPP4A, we hypothesized that increased calpain-protease-mediated degradation of INPP4A in mouse lungs may be important in experimental asthma pathogenesis. As an increase in the intracellular free calcium is known to activate the calpain family of proteases [30] , and abnormal calcium homeostasis has been observed in asthma [31] , [32] , it is very likely to be one of the underlying mechanisms for calpain-mediated INPP4A degradation. Various types of calpain inhibitors have been known to alleviate a myriad of disorders [33] , [34] . We selected calpeptin, as it was found to be the most potent among various calpain inhibitors, and also because of its potent cell penetrative nature in in vitro studies [35] . Importantly, calpeptin administration to mice with AAI restored activity and expression of INPP4A in bronchial epithelia ( Fig. 3d, e ). Calpeptin administration in this model of asthma also reduced the typical asthma-like features, such as AHR, infiltration of various inflammatory cells, including eosinophils in the bronchovascular region along with the reduction in IL-5 and other Th2 cytokines, goblet cell metaplasia and sub-epithelial fibrosis. Therefore, the restoration of INPP4A expression was associated with alleviation of asthmatic features. Loss of INPP4A in naive mice leading to development of AHR demonstrated the importance of INPP4A in pathogenesis of asthma ( Fig. 4 ). Dysregulation of the PI3K-Akt pathway due to reduced activity of INPP4A may lead to pathological consequences [36] as observed in this scenario ( Fig. 7 ). Although cellular infiltration was uncommon in INPP4A siRNA-treated naive mice, goblet cell metaplasia and sub-epithelial fibrosis were evident. There was a substantial increase in the activation of the PI3K-Akt signalling, which is the probable mechanism for increase in AHR, goblet cell metaplasia and collagen deposition, in line with existing evidence in which SHIP knock-out mice develop spontaneous allergic inflammation without any allergic sensitization and challenge [11] . To further confirm the protective role of INPP4A, we knocked down INPP4A by siRNA-mediated downregulation in mice with experimental asthma ( Fig. 5 ). Knockdown of INPP4A led to a worsening of the asthma phenotype, including severely increased airway inflammation, increased goblet cell metaplasia and increased airway remodelling. This was associated with accentuated PI3K-Akt signalling. We speculate that further knockdown of INPP4A in allergically inflamed lungs with low levels of INPP4A leads to loss of critical checkpoints on the PI3K-Akt signalling, and leads to a severe asthma phenotype. There is a growing body of evidence to suggest that PtdIns(3,4)P2 is critically required for the full activation of Akt as compared with PtdIns(3,4,5)P3, which further strengthens our observation [37] , [38] .Interestingly, inhibition of the PI3K signalling by wortmannin lead to partial restoration of INPP4A expression and resolution of airway inflammation ( Supplementary Fig. S8a-b ) in AAI models, possibly through some feedback mechanisms in the PI3K signalling cascade, which needs to be explored further. In support of a protective role of INPP4A in restricting airway inflammation and the asthma phenotype, we found that a gain-of-function approach by overexpression of INPP4A in the lungs of allergic mice would protect them from asthma. Intravenous administration of pCMV6-INPP4A plasmid using in vivo -jetPEI in the lungs of allergic mice led to attenuation of asthma phenotype, including AHR, airway inflammation and airway remodelling ( Fig. 6 ). There was no significant effect on histological goblet cell metaplasia in this model, possibly because of the patchy nature of overexpression. We are unable to exclude the possibility that reduced secretion of mucin, due to reduced cellular activation, may have counterbalanced any INPP4A overexpression-related direct reduction of mucin content of the airways. This is a technical limitation of the current methodology. 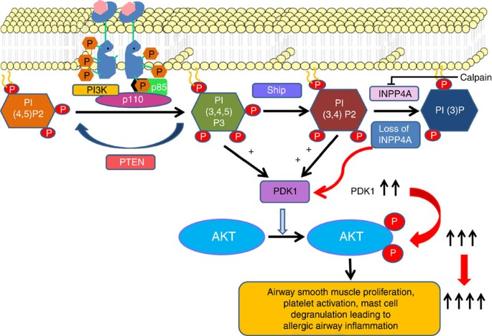Figure 7: Schematic model depicting the possible role of INPP4A in regulating the PI3K-Akt signalling in asthma. INPP4A dephosphorylates PtdIns(3,4)P2, and hence, inactivates the PI3K-Akt signalling. Calpain degrades INPP4A because of the presence of a PEST domain in INPP4A, and thus upregulates the PI3K-Akt signalling. Activation of Akt depends upon the phosphorylation of threonine and serine residues, which is catalysed by PDK1 (phosphoinositide-dependent kinase). Similar to Akt, PDK1 contains a PH domain and binds with high affinity to PtdIns(3,4)P2 (PI (3, 4)P2) and PtdIns(3,4,5)P3 (PI (3, 4, 5)P3, and thereby phosphorylate Akt. Binding of PtdIns(3,4)P2 to Akt causes a 3- to 5-fold stimulation of its activityin vitro, demonstrating the importance of PtdIns(3,4)P2 in activation of Akt, and thus the PI3K-Akt signalling. INPP4A being the terminal enzyme thus could more effectively regulate PI3K signalling. Hence, we propose that knockdown of INPP4A would lead to excess availability of PtdIns(3,4)P2 to PDK1, thereby resulting in increased levels of PDK1, which further leads to augmented activation of Akt, resulting in increased AAI. Figure 7: Schematic model depicting the possible role of INPP4A in regulating the PI3K-Akt signalling in asthma. INPP4A dephosphorylates PtdIns(3,4)P2, and hence, inactivates the PI3K-Akt signalling. Calpain degrades INPP4A because of the presence of a PEST domain in INPP4A, and thus upregulates the PI3K-Akt signalling. Activation of Akt depends upon the phosphorylation of threonine and serine residues, which is catalysed by PDK1 (phosphoinositide-dependent kinase). Similar to Akt, PDK1 contains a PH domain and binds with high affinity to PtdIns(3,4)P2 (PI (3, 4)P2) and PtdIns(3,4,5)P3 (PI (3, 4, 5)P3, and thereby phosphorylate Akt. Binding of PtdIns(3,4)P2 to Akt causes a 3- to 5-fold stimulation of its activity in vitro , demonstrating the importance of PtdIns(3,4)P2 in activation of Akt, and thus the PI3K-Akt signalling. INPP4A being the terminal enzyme thus could more effectively regulate PI3K signalling. Hence, we propose that knockdown of INPP4A would lead to excess availability of PtdIns(3,4)P2 to PDK1, thereby resulting in increased levels of PDK1, which further leads to augmented activation of Akt, resulting in increased AAI. Full size image As the PI3K signalling with consequent Akt phosphorylation can lead to the activation of a plethora of pathways that contribute to the pathogenesis of chronic disorders, such as asthma, INPP4A may serve as a regulatory checkpoint in the progression of asthma. Importantly, modulation of INPP4A without any intervention into the underlying immune disturbances was sufficient to modulate the asthma phenotype. Recent epidemiological and clinical data has suggested that the cardio-metabolic syndrome modulates asthma risk, severity and response to treatment [39] . Other than asthma, INPP4A has also been shown to be associated with cancer, acute myeloid leukemia and neuronal loss, suggesting that there may be important metabolic consequences of INPP4A dysregulation [40] , [41] , [42] . As increased PI3K signalling is also a feature of the metabolic syndrome, our findings offer novel insight into possible shared mechanisms, resulting in epidemiological associations between otherwise distinct diseases, such as asthma, hypertension, diabetes and so on. Indeed, there are recent reports that suggest a direct link between metabolic syndrome and asthma [39] , [43] . In conclusion, our results demonstrate for the first time that AAI in mice is associated with calpain-mediated degradation of INPP4A in the lungs, and that significant alleviation of asthma conditions were observed with restoration of INPP4A expression. Moreover, as deficiency of INPP4A in a normal lung can make the mice more susceptible for AHR, INPP4A could have a crucial role in maintaining epithelial homeostasis. Animals and grouping of mice Male BALB/c mice were maintained as per Committee for the Purpose of Control and Supervision of Experiments on Animals guidelines, and Institutional Animal Ethics Committee approved all protocols. There were six sets of mice: A, B, C, D, E and F. Set A had two groups (SHAM/PBS (saline controls), and OVA/OVA (OVA controls), ( n =8 each)); set B had three groups (SHAM/PBS, SHAM/Scrambled siRNA (8 mg kg −1 body weight) and SHAM/INPP4A siRNA (8 mg kg −1 body weight), ( n =6 in each)); set C had three groups ( Sham: SHAM/PBS/VEH, (VEH, vehicle was 1% dimethyl sulphoxide (DMSO)), OVA : OVA/OVA/VEH, Calpeptin : OVA/OVA/Calpeptin (0.05 mg kg −1 Calpeptin, Calbiochem, Germany); ( n =6 in each)) set D had four groups ( Sham: SHAM/PBS/VEH (vehicle was PBS), OVA: OVA/OVA/VEH, OVA/Scrambled siRNA : OVA/OVA/Scrambled siRNA (8 mg kg −1 ) and OVA/INPP4A siRNA : OVA/OVA/INPP4A siRNA (8 mg kg −1 ; n =6 in each)); and set E had three groups ( Sham : SHAM/PBS/VEH (vehicle was PBS), OVA/pCMV6 : OVA/OVA/pCMV6 (control vector, 50 μg, Origene, USA), OVA/pCMV6-INPP4A: OVA/OVA/pCMV6-INPP4A (50 μg, Origene; n =5 in each)). Set F had three groups: SHAM/PBS/VEH, OVA/OVA/VEH (DMSO as a vehicle), and OVA/OVA/WORT (WORT, wortmannin 0.1 mg kg −1 , Sigma Chemical Co., USA; n =5 in each). Sensitization and challenge of mice Mice were sensitized by three intraperitoneal (i.p.) injections of 50 μg OVA (OVA, chicken egg ovalbumin, Grade V, Sigma Chemical Co.) adsorbed in 4 mg alum to OVA groups or 4 mg alum alone to SHAM groups on days 0, 7 and 14. One week later, mice were challenged with 3% OVA aerosol (OVA groups) or PBS (SHAM groups) 30 min a day for 7 days consecutively, with a nebulizer (flow rate was 9 l min −1 , OMRON CX3 Model, Japan). siRNA and inhibitor delivery Calpeptin (0.05 mg kg −1 body weight) or DMSO was given i.p. to mice from day 21 to day 27, twice a day in a 200 μl volume per dose. INPP4A siRNAs (sense—5′-GGCUUUAUCAUCAAGCUGAdTdT-3′, antisense—5′-UCAGCUUGAUGAUAAAGCCdTdT-3′) were modified with 2′- O -methoxy at the 5′-end on both sense and antisense strands, and 'TT' dinucleotide overhangs were also incorporated to 3′-ends of siRNAs (Sigma Chemical Co). siRNAs were administered to normal and ova sensitized-challenged mice, using InExpose inhalation exposure system [44] ; pCMV6 and pCMV6-INPP4A was complexed with in vivo -jetPEI™ (Polyplus Transfection) in 400 μl of 5% glucose solution and injected into the tail vein. Two different concentrations of plasmids were initially chosen and given intravenously to mice. Wortmannin (0.1 mg kg −1 body weight per day) [45] was given i.p. on day 21, 23, 25 and 27 of ova challenge. Airway hyper-responsiveness Airway resistance was determined using the flexiVent (Scireq, Canada) invasive airway mechanics system [46] , [47] . Briefly, each mouse was anaesthetized with xylazine and pentobarbital sodium, intubated after tracheotomy and ventilated. Airway resistance was determined with administration of increasing concentrations of methacholine with nebulizer using the flexiVent system, which integrates the computer-controlled mouse ventilator with the measurements of respiratory mechanics. BAL and differential cell counts BAL was performed and differential cell counts were estimated [46] , [47] . Briefly, BAL was performed with cold PBS, centrifuged, and the cell pellets were resuspended in PBS, and cell smears were stained with Leishman stain to count at least 200 cells, to calculate the percentage of macrophage and mononuclear inflammatory cells, such as monocytes, neutrophils and eosinophils. Lung histopathology Lung sections were stained with haematoxylin and eosin, periodic acid-Schiff and Masson's trichrome stainings [46] . Briefly, one portion of the harvested lung was fixed with 10% buffered formalin. Paraffin-embedded lungs were cut into 5-ìμm sections and haematoxylin and eosin staining was performed to assess inflammatory changes, and stained sections were photographed with a Nikon microscope (Eclipse 90i) with camera. Slides were numbered randomly and evaluated blindly by two different investigators to determine inflammation scores. The quantity of perivascular or peribronchial inflammation was assessed as described previously [44] , with some modifications. Briefly, a grade of 0 was assigned when no inflammation was detectable, a grade 1 for occasional cuffing with inflammatory cells, and grades 2, 3 and 4 when most bronchi or vessels were surrounded by a thin layer (1–3 cells), a moderate layer (4–5 cells), a thick layer (more than 5 cells deep) of inflammatory cells, respectively. An increment of 0.5 was given if the inflammation fell between two grades. Total inflammation score was calculated by addition of both peribronchial and perivascular inflammation scores. Real-time PCR and flow cytometry Total RNA was extracted from control and allergic murine lungs, and siRNA-administered murine lungs (naive mice), according to manufacturer's protocol followed by real-time PCR [44] for INPP4A and glyceraldehyde 3-phosphate dehydrogenase (GAPDH). Real-time PCR oligonucleotide primer sequences were as follows: INPP4A: (sense): 5′-GTCCTCTTCAACGTGGGCATCAAT-3′; (anti-sense): 5′-TTTAACCGCACCAAGCTCTCCACA-3′; GAPDH: (sense): 5′-TCACCACCATGGAGAAGGC-3′. (anti-sense): 5′-GCTAAGCAGTTGGTGGTGCA-3′. Flow cytometry was performed with single-cell suspensions of the fresh lung. Briefly, lungs were harvested from control and allergic mice after it was killed, and mechanically disrupted with 70-μm cell strainer (Becton Dickinson, San Diego, CA, USA), red blood cells were lysed and removed with ACK lysis buffer (Invitrogen, USA) and stained with INPP4A and pan-Cytokeratin (1:50, C terminal antibody and 1:100, respectively; Cell Signalling Technology, USA) followed by acquisition and analysis using FACSCalibur [44] equipped with the Cell Quest software package (Becton Dickinson). Estimation of activities of INPP4A and calpain INPP4A activity was measured based on indirect estimation of PtdIns(3)P; briefly, lung cytosols were prepared using mitochondria isolation kit (MITO-ISO1, Sigma Chemical Co.) and were incubated (37 °C for 1 h) with 2 μM PtdIns(3,4)P2 (substrate of INPP4A) in reaction buffer [48] and reaction products were further incubated with PtdIns(3)P detector protein, followed by transferring final products to PtdIns(3)P-coated microplate for competitive enzyme-linked immunosorbent assay (ELISA), and the final INPP4A activity was expressed as PtdIns(3)P in picomoles produced from PtdIns(3,4)P2. Calpain activity was performed using a calpain activity assay kit (BIOvision, Inc., Mountain View, CA, USA). Enzyme-linked immunosorbent assay Levels of various cytokines ( IL-4 , IL-5 , IL-13 , IFN-γ and TGF-β1) , ova-specific IgE, IFN-α, IFN-β, IFN-γ, IL-12 and other mediators of the PI3K-Akt pathway ( INPP4A , pAkt Ser 473 , Akt kinase activity and PDK1) were measured as per respective manufacturer's protocols. Lung tissue homogenates were prepared by homogenizing 50 mg of the lung tissue in 500 μl PBS, followed by centrifugation at 10,000 g for 30 min and used for measuring different cytokines. The levels of mediators of the PI3k-Akt pathway were measured in lung cytosols. Cell line Human bronchial epithelial cells (BEAS-2B) were cultured with or without 20 ng ml −1 of recombinant IL-13 (R&D Systems, USA), and total lysates were prepared using RIPA buffer. INPP4A ELISA in primary murine airway epithelial cells Airway epithelial cells were isolated [49] followed by overnight pronase (Roche, USA) digestion and cultured in growth-factor-supplemented complete BEBM medium (Lonza, Switzerland), and induced with mouse recombinant IL-13 (R&D Systems) for 24 h, and total lysates were prepared using RIPA buffer for the estimation of INPP4A levels by ELISA (Uscn Life Science Inc., Wuhan, China). Immunohistochemistry Immunohistochemistry was performed [47] using goat polyclonal INPP4A primary antibody (1:75, Santa Cruz Biotechnology, USA) as primary antibody and horseradish peroxidase-conjugated anti-goat IgG (Sigma Chemical Co.) as secondary antibody. Goat gamma globulins (Jackson Immunoresearch Laboratories, Inc., USA) were used as isotype controls in negative control experiments. Immunoblotting Cytosolic extracts and total cell lysates were prepared from the mouse lung and cultured cells as per the manufacturer's instructions (Sigma Chemical Co). Proteins were separated on 8% SDS–polyacrylamide gel electrophoresis, transferred onto PVDF membranes (Millipore Corp., USA). Transferred membranes were blocked with blocking buffer (3% bovine serum albumin in Tris-buffered saline with Tween 20) for 1 h, and the blots were then probed with INPP4A (1:100, custom synthesized C terminus antibody), GAPDH (1: 1000, Santa Cruz Biotechnology), pAkt-Ser (1: 200, Santa Cruz Biotechnology), pAkt-Thr (1:200, Santa Cruz Biotechnology), Akt (1: 200, Santa Cruz) and α-tubulin (1:1000, Sigma Chemical Co.), detected with DAB-H 2 O 2 (Sigma Chemical Co.). Signals were detected by spot densitometry (Alpha EaseFC software from Alpha Innotech, CA, USA). Intravenous administration of plasmids using in vivo -jetPEI GFP-pCMV-INPP4A plasmid was complexed with in vivo -jetPEI and intravenously administered in mice. After 48 h of plasmid delivery, mice were killed, and images of the lung sections were taken using Leica macro confocal microscope (model TCS LSI 2, Leica, Germany) at ×1 and ×5 objective. Also, single-cell suspensions of fresh lungs were prepared, followed by acquisition for the green fluorescent protein expression and analysis using FACSCalibur [44] equipped with the Cell Quest software package (Becton Dickinson) were performed. In another group of mice, in vivo -jetPEI–FluoF (transfection regent labelled with fluorescein group (excitation and emission wavelength of 490 nm and 520 nm, respectively) was intravenously administered, mice were killed and images were captured as described earlier. Statistical analysis Significant differences between selected two groups were estimated using unpaired Student's t -test or post hoc testing, and Bonferroni correction for multiple corrections. Statistical significance was set at P ≤0.05. For knockdown experiments, one tailed t -test was used, as the experiments were based on a hypothesis and they are expected to turn out in a particular direction. How to cite this article: Aich, J., et al . Loss-of-function of inositol polyphosphate-4-phosphatase reversibly increases the severity of allergic airway inflammation. Nat. Commun. 3:877 doi: 10.1038/ncomms1880 (2012).